An OTX2-PAX3 signaling axis regulates Group 3 medulloblastoma cell fate OTX2 is a potent oncogene that promotes tumor growth in Group 3 medulloblastoma. However, the mechanisms by which OTX2 represses neural differentiation are not well characterized. Here, we perform extensive multiomic analyses to identify an OTX2 regulatory network that controls Group 3 medulloblastoma cell fate. OTX2 silencing modulates the repressive chromatin landscape, decreases levels of PRC2 complex genes and increases the expression of neurodevelopmental transcription factors including PAX3 and PAX6 . Expression of PAX3 and PAX6 is significantly lower in Group 3 medulloblastoma patients and is correlated with reduced survival, yet only PAX3 inhibits self-renewal in vitro and increases survival in vivo. Single cell RNA sequencing of Group 3 medulloblastoma tumorspheres demonstrates expression of an undifferentiated progenitor program observed in primary tumors and characterized by translation/elongation factor genes. Identification of mTORC1 signaling as a downstream effector of OTX2-PAX3 reveals roles for protein synthesis pathways in regulating Group 3 medulloblastoma pathogenesis. Brain tumors are the most deadly form of childhood cancer with medulloblastoma (MB) being the most common malignant primary pediatric brain tumor [1] . Despite numerous efforts to improve therapy, approximately one-third of MB patients die while survivors are left with lifelong neurocognitive sequelae, unable to live independent lives as a result of the toxicities associated with chemotherapy and radiation [1] , [2] . While historically considered a single disease, integrative genomic studies over the past decade have categorized MB into four highly distinct molecular subgroups: WNT, Sonic Hedgehog (SHH), Group 3, and Group 4 [1] , [3] , [4] , with further subclassification into multiple subtypes exhibiting distinct clinical outcomes [5] , [6] , [7] . Group 3 MB tumors represent a quarter of MB cases, display the worst prognosis, and are highly metastatic with over 50% of patients exhibiting tumor cell dissemination at diagnosis [2] . They are the most aggressive but the least understood in terms of tumor progression and developmental origins. While Group 3 MBs are believed to originate from either stem or/progenitor cell populations that exist transiently during early cerebellar development [7] , [8] , [9] , [10] , [11] , [12] , the molecular mechanisms that define these populations are not well understood. Cancer cells that adopt aberrant stem/progenitor cell signatures are associated with tumor propagation, metastasis, and drug resistance [13] . While targeted therapies are currently being evaluated in clinical trials (SJDAWN (NCT03434262) SJELIOT (NCT04023669) SJMB012 (NCT01878617)), further molecular characterization of the undifferentiated MB cells that harbor more primitive stem/progenitor signatures will undoubtedly lead to the development of additional treatment strategies that have less toxic effects on the developing nervous system. Orthodenticle homeobox 2 (OTX2) is a homeodomain transcription factor (TF) that plays pivotal roles in nervous system patterning, cell fate specification, and differentiation [14] , [15] , [16] . Mutations in OTX2 , particularly in the DNA-binding homeodomain, have been described in a number of brain and ocular defects [17] . Interestingly, amplification or increased expression of OTX2 is observed in over 80% of Group 3 and Group 4 MB [18] . Studies interrogating the function of OTX2 specifically in Group 3 MB have largely focused on its role in promoting tumor growth [19] , [20] , [21] . This has been attributed, at least in part, to a regulatory role for OTX2 in controlling the Group 3 MB chromatin landscape through association with active enhancer elements [22] , as well as maintenance of histone H3 lysine 27 trimethylation (H3K27me3) [23] . We have previously characterized a critical role for OTX2 in controlling cell fate decisions in Group 3 MB [24] , [25] . OTX2 silencing is accompanied by a robust increase in the expression of axon guidance genes, suggesting that OTX2 actively represses differentiation while maintaining Group 3 MB cells in a primitive, stem/progenitor cell state [25] . However, the majority of axon guidance genes identified were found to be indirect targets of OTX2 [25] . The mechanisms by which OTX2 inhibits differentiation of Group 3 MB cells are largely unknown. Thus, we sought to identify OTX2-binding partners and to further interrogate how OTX2 regulates genes associated with cell fate. Given the putative stem/progenitor cell of origin for Group 3 MB [26] , [27] , [28] , the disruption of H3K27me3 levels, as well as the presence of inactivating mutations in H3K27 demethylases in a subset of these tumors [29] , we posit that OTX2 plays a critical role in repressing a global differentiation gene signature in Group 3 MB. Thus, it is imperative to delineate the mechanisms by which OTX2 regulates MB tumor progression beyond cell proliferation and survival. In this study, we show that OTX2 broadly restricts expression of TFs that are critical for neuronal differentiation, including members of the PAX gene family. PAX genes play important roles in the developing nervous system, including the cerebellum [30] , [31] ; however, their specific effects on Group 3 MB progression have never been explored. PAX3 and PAX6 are epigenetically silenced in Group 3 MB patient samples and are direct targets of OTX2. Both PAX3 and PAX6 gain of function (GOF) results in decreased tumorsphere formation and SOX2 levels, as well as modulation of Group 3 MB gene signatures in vitro. However, only PAX3 overexpression reduces mTORC1 signaling and also increases survival in vivo. Finally, we define an OTX2-PAX3 gene regulatory network (GRN) that controls cell fate through mTORC1 signaling in highly aggressive Group 3 MB tumors. OTX2 regulates TF silencing in Group 3 MB To further investigate the role of OTX2 in regulating the chromatin landscape, we mapped genome-wide changes in activating (H3K4me3) and repressive (H3K27me3) histone modifications, following OTX2 silencing in stem cell-enriched D283 Group 3 MB tumorspheres (Fig. 1a ). We found that 8444 protein-coding genes displayed significant changes in H3K4me3 following OTX2 silencing, while 2001 genes had significant change in H3K27me3, and 564 genes showed changes in both histone marks (Fig. 1b, c ). Of the genes that exhibited a change in H3K4me3, 90% showed a significant gain in this activating histone mark, while 68% of genes with H3K27me3 changes displayed a significant loss of this repressive mark (Fig. 1d ). Overall, these findings suggest a global derepression of gene expression following OTX2 silencing in Group 3 MB. Fig. 1: PAX3 and PAX6 expression are reduced in Group 3 MB. a Workflow carried out to identify and characterize OTX2 target genes in Group 3 MB tumorspheres. b OTX2 silencing in D283 tumorspheres with two independent siRNAs after 24 h. β-actin serves as the loading control. c Number of protein-coding genes and transcription factors (TFs) with significant changes in H3K4me3 ( N = 8444 protein-coding genes, N = 419 TFs), H3K27me3 ( N = 2001 protein-coding genes, N = 144 TFs), and H3K4me3/H3K27me3 ( N = 564 protein-coding genes, N = 42 TFs) modifications following OTX2 silencing in D283 tumorspheres. d Proportion of protein-coding genes and TFs, with specific gain or loss of H3K4me3 or H3K27me3 modifications, respectively. e PAX3 (upper) and PAX6 (lower) expression analyses across the four medulloblastoma subgroups in two independent patient cohorts (MAGIC, N = 763 patient samples; Heidelberg, N = 167 patient samples) show lower PAX3 and PAX6 expression in Group 3 MB. The center line represents the median, the box represents the interquartile range, and the whiskers are the 95% confidence intervals. Data are presented as log2-transformed signal intensity. For the Heidelberg dataset, the outliers are defined as circles above and below the whiskers. Data are presented as log2-transformed signal intensity. For MAGIC cohort: PAX3 expression: all pairs *** p < 0.001 with the exception of Group 3 vs Group 4 * p < 0.05. PAX6 expression: all pairs *** p < 0.001 with the exception of WNT vs Group 4 NS. For Heidelberg cohort: 167 patients. PAX3 expression: all pairs *** p < 0.001 with the exception of Group 3 vs Group 4 NS. PAX6 expression: Group 3 vs Group 4 and Group 3 vs SHH *** p < 0.001. Group 4 vs SHH *** p < 0.001. SHH vs WNT ** p < 0.01. Group 3 vs WNT * p < 0.05. Group 4 vs WNT NS. Significance was determined by ANOVA with Tukey’s multiple comparisons. Full size image TFs play critical roles in neuronal specification, differentiation, and self-renewal during CNS development [32] . Therefore, we were interested in identifying TFs downstream of OTX2 that may belong to a larger OTX2-centric GRN controlling cell fate. Following OTX2 silencing, significant changes in H3K4me3 were identified in 419 TFs, changes in H3K27me3 were found in 144 TFs, and 42 TFs displayed changes in both modifications (Fig. 1c ). Interestingly, a greater proportion of TFs lost repressive histones modifications compared to protein-coding genes overall (Fig. 1d ), suggesting an important role for OTX2 in silencing TF expression in Group 3 MB tumorspheres. These TFs include a large number of genes belonging to the FOX, HOX, POU, PAX, SMAD, and SOX families (Supplementary Data 1 ). 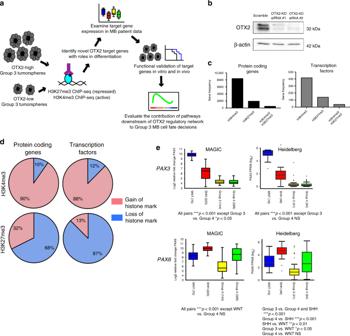Fig. 1:PAX3andPAX6expression are reduced in Group 3 MB. aWorkflow carried out to identify and characterize OTX2 target genes in Group 3 MB tumorspheres.bOTX2 silencing in D283 tumorspheres with two independent siRNAs after 24 h. β-actin serves as the loading control.cNumber of protein-coding genes and transcription factors (TFs) with significant changes in H3K4me3 (N= 8444 protein-coding genes,N= 419 TFs), H3K27me3 (N= 2001 protein-coding genes,N= 144 TFs), and H3K4me3/H3K27me3 (N= 564 protein-coding genes,N= 42 TFs) modifications following OTX2 silencing in D283 tumorspheres.dProportion of protein-coding genes and TFs, with specific gain or loss of H3K4me3 or H3K27me3 modifications, respectively.ePAX3(upper) andPAX6(lower) expression analyses across the four medulloblastoma subgroups in two independent patient cohorts (MAGIC,N= 763 patient samples; Heidelberg,N= 167 patient samples) show lowerPAX3andPAX6expression in Group 3 MB. The center line represents the median, the box represents the interquartile range, and the whiskers are the 95% confidence intervals. Data are presented as log2-transformed signal intensity. For the Heidelberg dataset, the outliers are defined as circles above and below the whiskers. Data are presented as log2-transformed signal intensity. For MAGIC cohort:PAX3expression: all pairs ***p< 0.001 with the exception of Group 3 vs Group 4 *p< 0.05.PAX6expression: all pairs ***p< 0.001 with the exception of WNT vs Group 4 NS. For Heidelberg cohort: 167 patients.PAX3expression: all pairs ***p< 0.001 with the exception of Group 3 vs Group 4 NS.PAX6expression: Group 3 vs Group 4 and Group 3 vs SHH ***p< 0.001. Group 4 vs SHH ***p< 0.001. SHH vs WNT **p< 0.01. Group 3 vs WNT *p< 0.05. Group 4 vs WNT NS. Significance was determined by ANOVA with Tukey’s multiple comparisons. The PAX gene family members PAX3 , PAX5 , PAX6 , PAX7 , and PAX9 all exhibited significant loss of H3K27me3, while PAX6 also showed significant gain of H3K4me3 (Table 1 ). The PAX family of TFs are critical for nervous system development [30] , [31] , yet their functional role in Group 3 MB pathogenesis has not been explored. Therefore, we focused our attention on the PAX genes for further study. Table 1 Derepression of PAX gene family members upon OTX2 silencing. Full size table Group 3 MBs exhibit low PAX3 and PAX6 expression We next evaluated transcript levels of the PAX genes exhibiting changes in histone marks, following OTX2 silencing across 763 subgrouped patient samples [5] . PAX3 and PAX6 were significantly lower in Group 3 and Group 4 MB relative to WNT and SHH MB tumors, while, PAX5 , PAX7 , and PAX9 were not significantly different between the four subgroups (Fig. 1e , Supplementary Fig. 1a–e ). PAX3 expression was remarkably high in WNT MB tumors that display the best overall prognosis [5] . Similar results were obtained for PAX3 and PAX6 in an independent MB patient sample cohort (Fig. 1e ), and are in stark contrast to the very high OTX2 levels observed in Group 3 and Group 4 MB [33] . Of note, PAX3 and PAX6 expression showed no significant correlation with MYC , which is highly expressed or amplified in Group 3 MB tumors (Supplementary Fig. 2 ) [34] , [35] . However, analyses of Group 3 MB clusters from patient sample single-cell RNA sequencing (scRNA-seq) data [11] revealed that OTX2 , while present in the majority of Group 3 MB cells, exhibited a wide range of expression (Fig. 2a, b ). Of note, PAX3 was not detectable in this dataset, and PAX6 was expressed at very low levels (Fig. 2b ). Interestingly, OTX2 expression is higher in clusters 9, 3, and 8 (Fig. 2b ). Clusters 9 and 3 correspond to clusters of cycling cells [11] , while cluster 8 consists of tumor cells expressing photoreceptor genes, such as CRX and RCVRN [11] . This is concordant with previous observations demonstrating that OTX2 expression is linked with cell cycle [19] , [21] , as well as photoreceptor genes [36] . Fig. 2: PAX3 and PAX6 protein levels are lower in Group 3 MB, and lower expression of both genes is associated with reduced survival in patients. a Nine transcriptionally distinct cell populations from two Group 3 MB patient samples as previously defined [11] . Of note, clusters 5, 10, and 11 were classified as non-tumor clusters and removed for downstream analysis. b Dot plot demonstrating the frequency and average expression of PAX6 (left) and OTX2 (right) within nine transcriptionally distinct cell populations from N = 2 Group 3 MB patient samples. Arrow denotes minimal expression of PAX6 in cluster 9. PAX3 was not detected in this dataset. c Low expression of both PAX3 and PAX6 is associated with significantly reduced overall patient survival in N = 612 MB patient samples. p -Values were determined using the log-rank method. d Representative images of PAX3 and PAX6 staining in FFPE sections from all four MB subgroups. Scale = 200 μm. e Proteomic analysis (Boston cohort) demonstrates low expression of PAX3 ( N = 27 patient samples) and PAX6 ( N = 45 patient samples) in Group 3 MB. For PAX3: WNT vs all other subgroups, *** p < 0.001, SHH vs Group 4: * p < 0.05, all other pairs NS. For PAX6: WNT vs SHH, * p < 0.05, SHH vs Group 3 and Group 4 *** p < 0.001, all other pairs NS. Significance was determined by one-way ANOVA. Full size image Analysis of the prognostic relevance of PAX3 and PAX6 revealed that higher expression was associated with significantly improved outcome (Fig. 2c ). In support of these findings, PAX3 and PAX6 levels were also lower in Group 3 formalin-fixed paraffin-embedded (FFPE) MB samples evaluated by immunohistochemistry (Fig. 2d ), as well as in a patient cohort recently characterized by proteomic analyses (Fig. 2e ) [37] , while OTX2 levels were very high in Group 3 MB tumors (Supplementary Fig. 3a ) [33] , [37] . As observed in the transcript data, PAX3 levels were highest in the WNT MB tumors, and PAX6 levels were elevated in the SHH MB subgroup (Fig. 2e , Supplementary Fig. 3b, c ). Interestingly, analyses of single-cell murine cerebellar transcript data ( https://cellseek.stjude.org/cerebellum ) [38] also revealed mutually exclusive expression patterns for Otx2 and Pax3 in a substantial number of cells, suggesting that a proportion of Otx2 + and Pax3 + cells have different developmental origins. Otx2 and Pax6 expression mainly overlap with the granule neurons/granule neuron progenitors defined by Atoh1 (Fig. 3a ) [39] . In contrast, Pax3 is mostly elevated in progenitors, some of which also express Ptf1a , a marker of early ventricular zone cells (Fig. 3a ) [39] , [40] . Thus, normal developmental expression patterns are somewhat divergent from those observed in MB. Collectively, our expression and survival analysis suggest that PAX3 and PAX6 may be associated with a more differentiated, less tumorigenic phenotype in Group 3 and Group 4 MB. Fig. 3: OTX2 directly regulates the expression of PAX3 and PAX6 in Group 3 MB. a Scatterhex plots showing expression of select genes obtained from https://cellseek.stjude.org/cerebellum/ . The gene expression of a hexgrid is summarized as the mean expression of all component cells and compared with predicted cell type mapped onto the scatterhex grid (upper left). b OTX2 enrichment is observed at regulatory elements on PAX3 and PAX6 , overlapping with H3K4me3 and H3K27me3 bivalency marks. c OTX2 binding to PAX3 and PAX6 was validated in D283, HDMB03, and MB3W1 Group 3 MB tumorspheres by ChIP-qPCR. Data are presented as mean values ± SEM. N = 3 biological replicates for each cell line. H3K4me3 ChIP-qPCR was used as a positive control. d Enrichment of H3K4me3, H3K27ac, and H3K27me3 at regulatory elements of OTX2 , PAX3 , and PAX6 , respectively, in five Group 3 MB patient samples as originally defined by Boulay et al. e Co-immunoprecipitation experiments showing protein–protein interaction between OTX2 and EZH2/SUZ12 in HDMB03 tumorspheres. CE cellular extracts. f EZH2 and SUZ12 levels are reduced following OTX2 silencing in D283, HDMB03, and MB3W1 tumorspheres. β-actin serves as the loading control. g PAX3 (left) and PAX6 (right) expression are significantly increased in Group 3 MB tumorspheres following OTX2 silencing for 72 h. Data are presented as mean values ± SEM and plotted as fold expression relative to scramble control. N = 3 biological replicates ( PAX3 expresion in HDMB03, PAX6 expression in D283, HDMB03); N = 4 biological replicates ( PAX3 expression in D283, MB3W1); or N = 5 biological replicates ( PAX6 expression in MB3W1). Significance was determined using an unpaired two-tailed t -test for each pair. For PAX3 : D283 p = 0.015; HDMB03 p = 0.005; MB3W1 p = 0.016. For PAX6 : D283 p = 0.005; HDMB03 p = 0.041; MB3W1 p = 0.023. h PAX3, but not PAX6 levels are increased following OTX2 silencing in D283 and HDMB03 tumorspheres. GAPDH serves as the loading control. Full size image OTX2 inhibits PAX3 and PAX6 expression in Group 3 MB Loss of H3K27me3 enrichment at PAX3 and PAX6 gene regulatory elements, following OTX2 silencing suggests that PAX3 and PAX6 expression are restricted by OTX2. To determine if OTX2 directly regulates PAX3 and PAX6 expression, we carried out OTX2 chromatin immunoprecipitation (ChIP)-sequencing in D283 tumorspheres. OTX2 enrichment at transcriptional start sites (TSS), and/or up/downstream gene regulatory regions was observed at PAX3 and PAX6 for D283 tumorspheres in situ (Fig. 3b ) . These areas of OTX2 enrichment overlapped with broad regions of H3K27me3 enrichment, while H3K4me3 enrichment was observed at the TSS of PAX3 and PAX6 , indicating a bivalency pattern, and overall transcriptional silencing (Fig. 3b ). Direct binding of OTX2 to PAX3 and PAX6 was validated by OTX2 ChIP-qPCR across three Group 3 MB cells lines (Fig. 3c ). We also interrogated a dataset containing five Group 3 MB patient samples to examine H3K27me3, H3K27ac, and H3K4me3 enrichment at PAX3 and PAX6 [22] . Broad H3K27me3 enrichment was observed at PAX3 and PAX6 across all five samples, with narrow H3K4me3 peaks at the TSS and negligible H3K27ac enrichment, consistent with our observations in D283 tumorspheres (Fig. 3d ). As expected, significant enrichment of H3K4me3, H3K27ac, and a lack of H3K27me3 were observed at OTX2 gene regulatory elements in association with high OTX2 levels in these tumors (Fig. 3d ). In addition to the direct binding of OTX2 to PAX 3 and PAX6 , we also examined whether OTX2 can interact with EZH2 and SUZ12. These proteins are members of the polycomb repressive complex 2 (PRC2) that establishes transcriptional silencing through trimethylation of histone H3 on lysine 27. Co-immunoprecipitation experiments revealed that OTX2 interacts with EZH2 and SUZ12 (Fig. 3e ). Interestingly, we also observed decreased EZH2 and SUZ12 levels following OTX2 silencing in tumorspheres (Fig. 3f ), suggesting that OTX2 can also regulate expression of these chromatin modifiers. Finally, significant reduction in H3K27me3 enrichment observed at PAX3 and PAX6 , following OTX2 silencing would suggest OTX2 restricts PAX gene expression in Group 3 MB. To confirm this, we carried out qPCR in D283, HDMB03, and MB3W1 Group 3 tumorspheres following OTX2 silencing. PAX3 and PAX6 expression were significantly increased in OTX2-silenced tumorspheres compared to controls (Fig. 3g ). Yet, only PAX3 sustained this increase at the protein level (Fig. 3h ). Collectively, these results demonstrate that OTX2 contributes to the epigenetic silencing of PAX3 and PAX6 expression in Group 3 MB. This occurs through multiple mechanisms, including direct binding of OTX2 to PAX3 and PAX6 , interaction with chromatin-modifying complexes, and regulation of EZH2 and SUZ12 levels. PAX3 significantly inhibits Group 3 MB properties PAX3 and PAX6 expression are directly repressed by OTX2 in Group 3 MB. Therefore, we hypothesized that increased PAX3 or PAX6 expression would reduce tumorigenic properties of OTX2 high Group 3 MB. To test this, we generated stable PAX3 and PAX6 GOF HDMB03 Group 3 MB cells (Fig. 4a, b ). PAX3 and PAX6 GOF inhibited tumorsphere formation compared to controls (Fig. 4c, d ). Upon passage to secondary tumorspheres, only PAX3 GOF tumorspheres sustained this significant decrease in sphere number, demonstrating a decrease in self-renewal capacity (Fig. 4c, d ). In addition, PAX3 GOF cells exhibited a 39% reduction in the frequency of cells in S phase, suggesting an inhibitory effect on proliferation (Fig. 4e, f ). No changes in the percentage of dead/dying cells were observed in PAX3 or PAX6 GOF (Fig. 4g, h ). Fig. 4: Increased PAX3 and PAX6 expression reduces tumorigenic properties of Group 3 MB cells. a , b PAX3 ( a ) and PAX6 ( b ) overexpression in HDMB03 Group 3 MB tumorspheres. GAPDH serves as the loading control. c , d Representative images ( c ) and quantification ( d ) of primary and secondary tumorspheres, with increased expression of PAX3 and PAX6. Error bars: SEM. Scale = 200 μm. N = 3 biological replicates for primary tumorspheres and N = 4 biological replicates for secondary tumorspheres. Significance was determined by ANOVA and a Tukey’s test for multiple comparisons. For primary tumorspheres: PAX3 GOF, p < 0.0001; PAX6 GOF, p = 0.0004. For secondary tumorspheres: PAX3 GOF, p = 0.023. e , f BrdU incorporation analysis in PAX3 and PAX6 GOF cells. Representative dot plot of gating strategy for BrdU analyses with 7AAD only control (inset) ( e ) and quantification of cell cycle phases in control, PAX3 GOF, and PAX6 GOF tumorspheres ( f ). Data are presented as mean values ± SEM. For PAX3 GOF “S” phase, p = 0.043. N = 4 biological replicates. g , h Annexin V/7AAD analyses of cell viability in PAX3 and PAX6 GOF cells. Representative dot plot of gating strategy for Annexin V/7AAD analyses ( g ) and quantification of live/dead cells in control, PAX3, and PAX6 GOF tumorspheres ( h ). Data are presented as mean values ± SEM. N = 3 biological replicates. For all flow cytometry data, signficance was determined by ANOVA followed by a Dunnett for multiple comparisons. i Increased PAX3 (upper) and PAX6 (lower) expression in HDMB03 cells utilized for intracerebellar transplants. GAPDH serves as the loading control. j Kaplan–Meier curves depicting overall survival in animals transplanted with 1 × 10 5 control, PAX3, or PAX6 GOF cells. p -Values determined using the log-rank method and p = 0.0014. k MRIs from two independent control and PAX3 GOF tumors (left) and H&E staining (right) from control and PAX3 GOF xenografts. Arrows denote tumors in the cerebellum. Scale = 400 μm. l Survival in xenografts transplanted with 2.5 × 10 4 control, PAX3, or PAX6 GOF cells. p -Values determined using the log-rank method and p = 0.040. m Representative images of Ki67, SOX2, and βIII tubulin levels in control, PAX3, and PAX6 GOF HDMB03 MB tumor-bearing mice. Scale bar: 100 μm. Full size image We next evaluated the effect of increased PAX3 and PAX6 expression on tumor growth in vivo. We first injected 1 × 10 5 PAX3 and PAX6 GOF HDMB03 cells into the cerebellum of NOD-SCID mice. Only PAX3 GOF animals displayed significantly increased survival compared to controls (Fig. 4 i, j ), and this was accompanied by a reduction in tumor size (Fig. 4k ). We repeated orthotopic injections using 2.5 × 10 4 cells per animal to further evaluate the tumor-initiating capacity of PAX GOF cells at lower doses. Increased survival in the PAX3 GOF was again observed compared to controls, while there was no significant change in PAX6 GOF (Fig. 4l ). This was not attributed to loss of PAX6 levels, as overexpression was sustained in vivo (Supplementary Fig. 4a ). Finally, in support of our tumorsphere assays, SOX2 was completely abolished in PAX3 GOF xenograft tumors, while small clusters of SOX2 were still evident in PAX6 GOF tumors (Fig. 4m ). Levels of the proliferation marker Ki67 were unchanged in both PAX3 and PAX6 GOF tumors (Fig. 4m ). Small increases in βIII tubulin levels were observed for PAX3 GOF tumors, while larger increases were evident in PAX6 GOF tumors. However, the βIII tubulin antibody is not human specific, and so to account for this issue, samples were also stained for the human marker STEM121 (Supplementary Fig. 4b ). While all tumors are strongly and homogeneously STEM121 positive, we cannot rule out the possibility that some of the βIII tubulin staining, particularly at the tumor/mouse brain interface may represent contributions from mouse cells. Collectively, these results demonstrate that PAX3 is a potent inhibitor of neoplastic properties in vitro and, on its own, is sufficient to enhance Group 3 MB survival and abolish SOX2 levels in vivo. PAX3 uniquely modulates mTORC1 signaling pathway genes To delineate the molecular mechanisms that distinguish the effects of PAX3 and PAX6 GOF Group 3 MB cells, we performed RNA-seq on PAX3 and PAX6 GOF HDMB03 tumorspheres (Fig. 5a , Supplementary Fig. 5a ). We identified 1564 and 1542 differentially expressed genes in PAX3 GOF and PAX6 GOF tumorspheres, respectively (Fig. 5b, c ). The majority of differentially expressed genes were uniquely upregulated or downregulated in PAX3 or PAX6 GOF tumorspheres (71.99% in PAX3 GOF, 71.59% in PAX6 GOF). However, 186 genes were upregulated and 182 genes were downregulated in both PAX3 and PAX6 GOF tumorspheres. Gene set enrichment analysis (GSEA) revealed that gene sets associated with GABA and glutamate receptor activation, as well as PKCA signaling were enriched for genes that are downregulated in PAX3 and PAX6 GOF tumorspheres (Fig. 5d ). In contrast, gene sets associated with photoreceptor signaling are enriched for genes that are commonly upregulated in PAX3 and PAX6 GOF tumorspheres. Interestingly, GABAergic, glutamatergic, as well as photoreceptor molecular signatures are typically associated with Group 3 and/or Group 4 MB [4] , [41] , thus providing validation for the use of tumorspheres as surrogate models for studying pathways regulating MB progression. In support of these findings, gene ontogeny and KEGG pathway analyses demonstrated that GABAergic and glutamatergic transmitter-gated ion channel genes were differentially expressed in both PAX3 and PAX6 GOF (Supplementary Fig. 5b ). Epithelial cell proliferation and stem cell genes, including CCND1 and SOX2 were similarly downregulated in both PAX3 and PAX6 GOF tumorspheres (Supplementary Fig. 5c ). Expression of a number of axonal guidance genes was also significantly changed in both PAX3 and PAX6 GOF cells. For example, EPHB2 was significantly upregulated in both cell populations, while EPHB3 was uniquely upregulated in PAX3 GOF (Supplementary Fig. 5d ). Fig. 5: PAX3 and PAX6 expression perturb Group 3 transcriptional signatures. a Increased expression of PAX3 and PAX6 in Group 3 HDMB03 PAX3 and PAX6 GOF tumorspheres validated at the transcript level by RNA sequencing. b Volcano plots depicting fold changes of differentially expressed genes identified in PAX3 (1564) and PAX6 (1542) GOF tumorspheres. * p < 0.05 for all genes. c Venn diagram comparing unique and shared upregulated or downregulated genes identified to be differentially expressed in PAX3 and PAX6 GOF HDMB03 tumorspheres. * p < 0.05 for all genes. d GSEA demonstrating that GABA receptor activation, as well as glutamate and PKCA signaling are enriched in gene sets that are downregulated in PAX3 and PAX6 GOF tumorspheres. Genes associated with photoreceptor signaling are enriched in gene sets that are commonly upregulated in PAX3 and PAX6 GOF tumorspheres. e mTORC1 signaling is enriched in gene sets that are downregulated in PAX3 GOF tumorspheres. Genes associated with MYC targets are enriched in PAX6 GOF tumorspheres. f Normalized cell counts from RNA sequencing data showing decreased SOX2 , and increased TUJ1 (βIII tubulin) or EPHB2 in PAX3 and/or PAX6 GOF tumorspheres. g Validation of changes in SOX2, βIII tubulin, EPHB2, and DCX levels in PAX GOF tumorspheres. β-actin and GAPDH serve as loading controls. h Reduction in overall mTORC1 activity output observed specifically in PAX3 GOF tumorspheres. Total S6, total 4E-BP1, total Raptor, and β-actin serve loading controls. Note that for all RNA sequencing data, significantly different genes were identified using a q -value (Benjamini–Hochberg corrected p -value) cutoff of 0.05. Full size image In addition to the differentially expressed genes in both PAX3 and PAX6 GOF cells, GSEA also identified pathways that could be uniquely contributing to the in vitro and in vivo properties for each cell type. The MSigDB mTORC1 signaling hallmark gene set is significantly enriched only for genes downregulated in PAX3 GOF, while the MYC target hallmark gene list is enriched in genes upregulated in PAX6 GOF tumorspheres (Fig. 5e , Supplementary Data 2 , 3 ). We next validated differentially expressed genes, and pathways associated with neuronal differentiation and self-renewal by immunoblot. In support of our xenograft data in Fig. 4m , the stem cell marker SOX2 was undetectable in PAX3 GOF, but still present in PAX6 GOF tumorspheres (Fig. 5f, g ). Similar to our in vivo data, the neuronal lineage markers doublecourtin (DCX) and βIII tubulin ( TUJ1 ) were markedly upregulated only in PAX6 cells. Interestingly, the axon guidance neurodevelopmental gene EPHB2 was increased in both PAX GOF tumorspheres (Fig. 5f, g ), suggesting that PAX3 and PAX6 have variable effects on stem cell and differentiation genes. As PAX3 GOF cells showed more prominent effects on tumorigenic properties, mTORC1 activity was further evaluated. mTORC1 signaling is associated with regulation of protein synthesis, and this is mediated through the phosphorylation of eukaryotic translation initiation factor 4E-binding protein 1 (4E-BP1) and S6 ribosomal protein [42] . A reduction in mTORC1 signaling activity, as measured by p-S6 and p-4E-BP1, was observed only in PAX3 GOF tumorspheres (Fig. 5h ). Similarly, a decrease in the upstream mTORC1 regulator, Ras homolog enriched in brain (RHEB) is only observed in PAX3 GOF tumorspheres, while pRaptor, a component of the mTORC1 complex, is increased in PAX3 GOF cells (Fig. 5h ). Collectively, these results demonstrate that PAX3 and PAX6 induce changes in Group 3 MB transcriptional signatures. However, PAX3 uniquely abolishes SOX2 levels and regulates mTORC1 signaling outlining a potential pathway through which this TF specifically contributes to self-renewal of Group 3 MB cells. mTORC1 signaling is associated with a stem cell program Our results show an inverse correlation between PAX3 expression and mTORC1 activity in Group 3 MB tumorspheres. However, tumorspheres are heterogeneous populations of stem cells, progenitors, and more differentiated neural progeny. Therefore, we performed scRNA-seq on tumorspheres derived from three Group 3 MB cell lines to determine whether analogous expression patterns are observed at the individual cell level. Analyses of three Group 3 MB cell lines revealed individual clusters marked by cell cycle genes and histones (Supplementary Fig. 6a–c , Supplementary Data 4 ). OTX2 expression patterns were similar to those observed for Group 3 MB patient tumors (Fig. 2a, b ), in which OTX2 is variably expressed but is at least detectable in the majority of cells across all three tumorsphere populations. Similarly, the mTORC1 genes, EIF4EBP1 / RPS6 , were variably expressed across the transcriptionally distinct clusters, while PAX gene expression was negligible or absent throughout (Supplementary Fig. 6d–f ). We used the three metaprograms described by Hovestadt et al. [12] from Groups 3 and 4 (Group 3/4-A, Group 3/4-B, Group 3/4-C) representing cycling, undifferentiated, and differentiated transcriptional programs and evaluated their relative expression across our Group 3 tumorspheres. The undifferentiated “metaprogram” is characterized by ribosome and translation/elongation factor genes [12] and is associated with a high metascore across the transcriptionally distinct clusters for all three tumorsphere populations. Interestingly, correlation plots demonstrate that the undifferentiated program is negatively correlated with cell cycle, while it is positively correlated with genes associated with protein synthesis/translation initiation and ribosome biogenesis (Supplementary Fig. 6g–i , Supplementary Fig. 7a, b ). In the Hovestadt et al. study, almost 90% of Group 3 MB tumor cells are associated with this undifferentiated cell metaprogram. In contrast, a neuronal-differentiated metaprogram was dominant in almost all Group 4 MB tumor cells [12] . Thus, the undifferentiated metaprogram and the ribosomal and translation initiation/elongation genes associated with it are subgroup specific. To gain further insight into the cell identity of transcriptionally distinct clusters and the association of mTORC1 signaling with these clusters, scRNA-seq data from all three sets of tumorspheres were integrated (Fig. 6a–c ). Similar to the results from individual cell lines, a negative correlation between the undifferentiated program and cell cycle, as well as a positive correlation between the undifferentiated program and translation initiation (Fig. 6d, e ) were observed. Moreover, a positive and negative correlation were also observed between the undifferentiated program and our mTORC1 gene signature, and cell cycle and our mTORC1 gene signature, respectively (Fig. 6f, g ). These findings prompted a more thorough examination of individual cluster identity. While it was difficult to annotate cellular identity for all the clusters, we observed high expression of Nestin ( NES ), a neural stem cell marker in cluster 3. In addition, clusters 1, 2, and 4 express the more differentiated unipolar brush cell marker Eomesodermin ( EOMES ; Fig. 6h, i ). Clusters 3 and 4 appear to have the lowest cycling score across clusters with cluster 4 representing a more differentiated phenotype (Fig. 6j ). Importantly, translation initiation as well as our overlapping, but more context-specific mTORC1 gene signature are broadly expressed across all clusters, but are highest in the lower-cycling NES + cell compartment (Fig. 6j ). Fig. 6: Integrated scRNA-seq analyses of Group 3 tumorspheres reveals relationships between the undifferentiated stem/progenitor cell state and an mTORC1 gene expression signature. a – c UMAP representations of integrated tumorsphere data from D283, HDMB03, and MB3W1 ( a ), cell cycle phases from integrated data ( b ), and transcriptionally distinct cell populations from integrated data ( c ). d – g Correlation plots displaying the relationship between the undifferentiated program and cell cycle ( d ), as well as the undifferentiated program and translation initiation ( e ), the undifferentiated program and our mTORC1 gene signature ( f ), and cell cycle and our mTORC1 gene signature ( g ) from integrated tumorsphere data. The mTORC1 gene signature overlaps with the broad translation initiation program, but is based on the curated list of genes provided in Supplementary Data 8 , the majority of which  are associated with the 4E-BP1 and S6 ribosomal protein arms of mTORC1 signaling, and are also direct OTX2 targets. h , i Expression of the neural stem cell marker Nestin ( NES ) and the differentiated unipolar brush cell marker Eomesodermin ( EOMES ) in clusters of the integrated tumorsphere data. j Expression of the cell cycle, undifferentiated, differentiated, and translation initiation programs, as well our mTORC1 gene expression signature across clusters in the integrated tumorsphere data. For the three biologically independent cell lines, n = 6307 cells (HDMB03), n = 5297 cells (D283), and n = 5099 cells (MB3W1). For all violin plots, the center line is the median, the 25th and 75th percentiles are depicted by the bottom and top of the box, respectively, and the whiskers extend to the minima and maxima. Full size image Collectively, our individual cell line and integrated scRNA-seq data demonstrate that protein synthesis pathway activities and more specifically our mTORC1 gene signature are associated with undifferentiated stem/progenitor Group 3 MB cell populations. These findings provide support for the notion that mTORC1 signaling is a component of a self-renewal program regulating Group 3 MB cell fate. OTX2 silencing in Group 3 MB cells reduces mTORC1 activity Increased PAX3 expression has similar functional consequences to OTX2 silencing, including reduced self-renewal and proliferation [24] , [25] . Therefore, we predicted that OTX2 silencing would also decrease mTORC1 activity. We first examined the pathways that were associated with genes that had significant changes in H3K4me3 and H3K27me3 upon OTX2 silencing in D283 tumorspheres. Genes involved with the regulation of eukaryotic initiation factor 2 (EIF2) signaling, mTORC1 (eIF4 and p70S6K (p-S6)), or mTOR signaling in general exhibited significant changes in H3K4me3 only (Fig. 7a–c , Supplementary Data 5 – 7 ). Additional analyses demonstrated that many mTORC1-related genes also exhibit OTX2 peaks and motifs, indicating that they could be directly regulated by OTX2 (Supplementary Data 8 ). Interestingly, these specific OTX2-binding peaks do not contain PAX3 motifs (Supplementary Data 8 ), suggesting that PAX3 may regulate mTORC1 genes at different regulatory elements. Our pathway analysis on the altered histone landscape demonstrates that genes central to mTORC1 display significant changes at the epigenome level following OTX2 silencing. Fig. 7: Loss of OTX2 phenocopies PAX3 and PAX6 GOF in Group 3 MB cells. a – c EIF2 and mTORC1 signaling (highlighted) associated with genes that have significant changes in the H3K4me3 modification, following OTX2 silencing in Group 3 MB tumorspheres. Significance was calculated using a right-tailed Fisher’s exact test. d , e OTX2 silencing in HDMB03 ( d ) and D283 ( e ) tumorspheres with two independent siRNAs reduces SOX2, p-S6, p-4E-BP1, and Rheb levels. The neuronal differentiation markers DCX, βIII tubulin, and EPHB2 are increased along with small increases in pRaptor in D283 tumorspheres only. Total S6, total 4E-BP1, total Raptor, GAPDH, and β-actin serve as loading controls. f Enriched biological processes and pathways determined using GSEA (Terms with FDR corrected q -value < 0.25) and visualized in Cytoscape v3.7.2 using Enrichmentmap. Each node in the map denotes a pathway, process or a transcription factor enrichment. The size of the nodes is proportional to the number of genes in the process. The nodes are connected when they share enriched genes. Nodes with asterisk denote the processes enriched with q < 0.05. g Representative images of p-S6 and p-4E-BP1 immunohistochemical staining in three independent FFPE Group 3 (upper) and Group 4 (lower) MB patient samples. Scale = 200 μm. Full size image To validate these findings, we silenced OTX2 expression in Group 3 MB tumorspheres and examined mTORC1 activity. OTX2 silencing in HDMB03 and D283 tumorspheres resulted in decreased SOX2, and/or increased DCX and βIII tubulin (Fig. 7d, e ). This was accompanied by an overall decrease in mTORC1 activity, as depicted by lower p-S6, p-4E-BP1, and RHEB (Fig. 7d, e ) levels. A small increase in pRaptor was only observed following OTX2 silencing in D283 tumorspheres. Collectively, these results demonstrate that OTX2 silencing phenocopies the reduction in mTORC1 activity observed in PAX3 GOF tumorspheres, and suggests that this pathway is intimately linked with the stem cell/progenitor phenotype in Group 3 MB. mTORC1 activity regulates Group 3 MB tumor properties The unique downregulation of mTORC1 signaling in PAX3 GOF tumorspheres could be a potential mechanism contributing to reduced self-renewal capacity, as well as the increased survival observed in the PAX3 GOF animals. We therefore decided to evaluate the effects of dual mTORC1/2 inhibitors in Group 3 MB, as mTORC1-specific inhibitors have largely failed in the clinic due, in part, to released inhibition of mTORC2/AKT signaling upon blocking mTORC1 [42] . We first performed pathway enrichment analyses using gene expression data from 763 MB patient samples [5] to determine whether protein synthesis and/or mTORC1 pathway genes were upregulated in Group 3 MB tumors. Indeed, rRNA processing, ribosome maturation, and activation, translation initiation, translation, and posttranslational protein targeting along with MYC-related genes [5] were upregulated in Group 3β and 3γ compared to all other MB subtypes (Fig. 7f ). Notably, the gene targets of the TF cone-rod homeobox (CRX), which is activated by OTX2 [43] , were also enriched in Group 3β and 3γ MB. We also examined mTORC1 activity in Group 3 MB FFPE tumor sections. Group 3 MB patient samples exhibit a range of positive p-S6 and p-4E-BP1 staining (Fig. 7g ). Group 4 MB tumors, which also have high OTX2 expression, exhibit p-S6 (Fig. 7g ), albeit to a lesser extent in a small subset, as well as a range of positive p-4E-BP1 staining (Fig. 7g ), suggesting that cells with active mTORC1 signaling are a therapeutically targetable cell population in both MB subgroups. Next, we assessed the efficacy of two dual mTORC1/2 inhibitors: AZD8055 as well as the drug PQR620 in Group 3 MB tumorspheres. After 3 h treatment, a striking reduction in p-S6 was observed for AZD8055, while only a small inhibition of p-AKT (mTORC2) was evident at higher concentrations (Fig. 8a ). Treatment with PQR620 also resulted in a dose-dependent reduction in p-S6, but had negligible effects on p-AKT after 24 h (Fig. 8b ). Therefore, in our Group 3 MB models, both drugs have a more pronounced effect on mTORC1 activity. Interestingly, we observed decreases in EZH2 levels following AZD8055 and, to a lesser extent, PQR620 treatment at the higher concentrations (Fig. 8a, b ), suggesting that mTOR signaling can also modulate PRC2 complex protein levels in MB. Fig. 8: mTORC1 signaling regulates tumorsphere formation and self-renewal in Group 3 MB. a , b mTOR signaling and EZH2 levels following 3 h AZD8055 ( a ) or 24 h PQR620 ( b ) treatment in Group 3 MB tumorspheres. Total S6, total AKT, and β-actin serve loading controls. c Representative H&E as well as immunohistochemical images of STEM121, Ki67, SOX2, and βIII tubulin levels in control and PQR620-treated HDMB03 tumor-bearing NOD-SCID mice 14 days postinjection. Scale bars: 1000 μm (H&E and STEM121) or 100 μm (Ki67, SOX2, βIII tubulin). d Survival in animals transplanted with 1 × 10 5 cells from HDMB03 tumorspheres and treated with vehicle ( N = 17) or PQR620 ( N = 10 50 mg/kg, and N = 9 100 mg/kg). p -Value determined using the log-rank method. p = 0.0001 for 50 mg/kg and p = 0.002 for 100 mg/kg. e Representative images of tumorspheres following AZD8055 treatment of HDMB03 Group 3 MB cells. Scale = 200 μm. f Quantification of total sphere number (upper) and viability (lower) following HDMB03 Group 3 tumorsphere treatment with AZD8055. Error bars: SEM. N = 3 biological replicates. For total sphere number: p = 0.0035 (0.25 μM); p = 0.0014 (0.5 μM); p = 0.0007 (2.0 μM). For viability: p < 0.0001 for all concentrations. g Representative images of tumorsphere number following HDMB03 PQR620 treatment. Scale = 200 μm. h Quantification of total sphere number (upper) and viability (lower) following HDMB03 treatment with PQR620. N = 4 biological replicates. For total sphere number: p = 0.038 (10 μM). i , j Quantification of primary ( i ) and secondary ( j ) HDMB03 tumorsphere number, and viability following AZD8055 treatment (25–100 nM). For primary sphere number: p = 0.002 (0.025 μM); p < 0.0001 for remaining concentrations. For viability: p = 0.0362 (0.05 μM); p = 0.0002 (0.1 μM). For secondary sphere number: p = 0.043 (0.1 μM). For viability: p = 0.035 (0.05 μM); p = 0.0004 (0.1 μM). k Western blots depicting SOX2, βIII tubulin, and cleaved caspase 3 levels, following AZD8055 (upper) or PQR620 (lower) treatment of HDMB03 tumorspheres at 24–72 h. GAPDH serves as the loading control. For all tumorsphere studies, data are presented as mean values ± SEM, and significance was determined by one-way ANOVA and a Dunnett test for multiple comparisons. l Model demonstrating an OTX2-PAX3 circuitry regulates cell fate decisions through control of mTORC1 signaling. Full size image PQR620 [44] , unlike AZD8055 [45] , has been shown to cross the blood–brain barrier. Thus, we also examined the effects of PQR620 treatment in vivo. Tumor-bearing NOD-SCID mice treated with PQR620 exhibited dramatic decreases in tumor growth (Fig. 8c ). Similar to PAX3 GOF tumors in vivo, PQR620-treated tumors also exhibit decreased SOX2, as well as increased βIII tubulin levels (Fig. 8c ). As observed in PAX GOF tumors, the main tumor mass is STEM121 positive; however, we cannot rule out the possibility that a proportion of βIII tubulin staining represents contributions from infiltrating mouse cells, particularly at the tumor/mouse brain boundary (Fig. 8c , Supplementary Fig. 8a ). In addition, Ki67 levels are minimally decreased following treatment (Fig. 8c ). These phenotypic changes were also accompanied by a significant increase in survival (Fig. 8d ). Collectively, these results demonstrate that PQR620 significantly reduces tumorigenic properties in a highly aggressive Group 3 MB xenograft model. To further delineate the potential role for these inhibitors in cell fate decisions, we evaluated the effects of AZD8055 and PQR620 on tumorsphere formation and self-renewal. AZD8055 treatment significantly inhibited or completely abolished Group 3 MB tumorsphere formation respectively, while increasing cell death (Fig. 8e, f , Supplementary Fig. 8b, c ). Similar results were obtained for PQR620 treatment, albeit to a lesser extent (Fig. 8g, h , Supplementary Fig. 8d, e ). As some tumorsphere formation was retained following HDMB03 treatment with AZD8055, we repeated these studies using a lower concentration range (25–100 nM) to enable generation of secondary tumorspheres and assessment of self-renewal (Supplementary Fig. 8f–h ). Indeed, AZD8055 inhibited HDMB03 self-renewal (Fig. 8i, j , Supplementary Fig. 8g, h ) and this was also associated with decreased SOX2 levels (Fig. 8k , upper). Similar to PAX3 GOF tumorspheres, we did not observe an increase in βIII tubulin at sublethal concentrations (Fig. 8k , upper). The same patterns were observed for PQR620 (Fig. 8k , lower), in which SOX2 was strongly decreased, while βIII tubulin did not change at lower concentrations. Collectively, these results demonstrate that mTOR signaling regulates stem cell properties in Group 3 MB. Studies examining the role of OTX2 in Group 3 MB progression have mainly focused on the epigenetic and transcriptional activation of cell cycle genes [19] , [20] , [21] , [22] . We have shown that this multifaceted TF is a broad regulator of genes associated with protein synthesis in Group 3 MB. The downstream effect on mTORC1 signaling may be regulated either directly by OTX2 or indirectly through modulation of PAX gene expression (Fig. 8l ). This circuitry may control key cell fate decisions in Group 3 MB stem/progenitor cells, thus expanding the scope of OTX2’s regulatory role in MB pathogenesis. A previous study evaluated the role of OTX2 in regulating H3K27me3 modifications in Group 3 MB [23] . However, following OTX2 silencing, the authors reported no overall expression changes in the majority of genes that lost H3K27me3 and were bound by OTX2. In contrast, we identified genes whose predicted changes in histone marks are correlated with changes in gene expression. When OTX2 was downregulated, we observed significant increases in PAX3 and PAX6 expression. For PAX3, this increase was also sustained at the protein level. Moreover, both genes are direct transcriptional targets of OTX2 and display significant reduction in H3K27me3 following OTX2 silencing. It’s worth noting that in the previous study by Bunt et al., a small percentage of genes were found to have an overall up/downregulation in gene expression following OTX2 silencing [23] . It would be interesting to evaluate whether these genes are also associated with protein synthesis pathways. In addition, our data also suggest that OTX2 plays a much larger role in regulating TF expression. Direct binding to genes, such as PAX3 and PAX6 , interaction with chromatin-modifying complexes, and regulation of EZH2 and SUZ12 expression are all mechanisms by that OTX2 may suppress neural differentiation. We determined that PAX3 and PAX6 expression are correlated with increased survival in patient samples, and are directly repressed by OTX2 in Group 3 MB. In particular, PAX3 overexpression significantly inhibited Group 3 tumorigenic properties in vitro, while increasing survival in our intracerebellar transplant models. Interestingly, this is in contrast to the role of PAX3 in other brain tumors, where it has been shown to be oncogenic in glioblastoma [46] , thus underscoring the cell context-dependent role of PAX TFs in neural cancers. The PAX gene family coordinate a myriad of developmental programs, including self-renewal and neuronal differentiation [30] . While PAX6 has been shown to specifically control the balance between neural stem cell self-renewal and differentiation [47] , very little is known about how PAX3 regulates these processes. Both PAX3 and PAX6 differentially affect Group 3 MB cell fate in vitro; however, OTX2-PAX3 specifically modulates mTORC1 signaling. Moreover, PAX3, on its own, was sufficient to enhance survival in vivo. Thus, PAX3 and PAX6 are not functionally redundant in Group 3 MB. We have recently begun to appreciate how neurodevelopmental programs are hijacked during Group 3 MB progression [36] . These highly aggressive tumors are associated with several molecular signatures [3] , [4] , [36] , including GABAergic and glutamatergic signaling, as well as a photoreceptor differentiation program. Our RNA-seq results demonstrated that these Group 3 MB signatures were all enriched in gene sets that were either upregulated or downregulated in PAX3 and PAX6 GOF HDMB03 tumorspheres. Moreover, our scRNA-seq data revealed enrichment of an undifferentiated progenitor program that is widely expressed in Group 3 MB patient samples [12] and is characterized by genes associated with protein synthesis. These results highlight the strength of our tumorsphere models in dissecting pathways directly relevant to primary Group 3 MB samples. Our multiomics data and subsequent proof of principle studies with AZD8055 and PQR620 provide a rationale for targeting treatment resistant Group 3 MB stem/progenitors through inhibition of mTOR signaling. Dual PI3K/mTOR inhibitors have previously been shown to be effective in the treatment of MYC-amplified genetically engineered Group 3 MB mouse models [26] , [48] . However, to our knowledge, a specific role for mTORC1 signaling as a regulator of human Group 3 MB cell fate has not previously been reported. The results from this study demonstrate that OTX2 plays a much more comprehensive role in Group 3 MB progression than previously appreciated. Further exploration of OTX2’s position within the highly heterogeneous MB neural lineage cellular hierarchy may reveal divergent and even more complex roles in MB cell fate decisions and metastasis. For example, both OTX2 and PAX3 are highly expressed in WNT MB tumors. As the WNT subgroup has very good overall prognosis compared to Group 3 MB, the functional contribution of OTX2 is clearly subgroup dependent. This will be particularly important, as our analyses of single-cell murine cerebellum data suggested that Otx2 + and Pax3 + cells may have different developmental origins. While rare, OTX2 expression has also been observed in a small subset of human SHH samples [33] . Additional studies will therefore be required to better understand the biology of all OTX2+ lineages, further delineate their transcriptomes, and to determine how they are mirrored or diverge from Group 3 MB. This will lead to the identification of additional key molecular players that can be further exploited therapeutically to treat these highly aggressive tumors. Cell culture and in vitro drug treatments The D283 [49] cell line was purchased from the American Type Culture Collection (ATCC, Rockville, MD, USA). The HDMB03 Group 3 MB cell line was a kind gift from Dr. Till Milde [50] . Dr. Matthias Wölfl kindly provided the recently derived MB3W1 Group 3 cell line [51] . STR profiling (ATCC) was used to authenticate all cell lines utilized in this study. D283 tumorspheres were prepared in Neural Precursor media [24] (Life Technologies, Burlington, ON, Canada) and cultured in ultra-low-attachment plates. HDMB03 and MB3W1 tumorspheres were prepared in StemPro NSC Serum-Free Medium (Life Technologies) and Stem Cell Media (DMEM/F12, 2% B27, 1% MEM vitamin solution, 20 ng/mL bFGF, 20 ng/mL EGF, 40 U/ml penicillin, and 40 μg/ml streptomycin), respectively, on ultra-low-attachment plates. For tumorsphere assays, cells were plated at clonal density (D283: 5 cells/μl, HDMB03: 2.5 cells/μl, MB3W1: 5 cells/μl) in 24-well ultra-low-attachment plates. For tumorspheres assays with mTOR inhibitor treatment, AZD8055 (Selleckchem, Houston, TX, USA) was added at 10 nM–2.0 μM, and PQR620 (MedChemExpress, Monmouth Junction, NJ, USA) was added at (2–100 μM) at day 0, following by 5 days incubation at 37 °C, 5% C0 2 . For in vitro validation of mTOR inhibitors, 2 × 10 5 cells/well were plated in the drug concentrations described above for 3 h prior to collection and evaluation by western blot. ChIP and sequencing Group 3 MB cells were plated in stem cell conditions and cultured for 3 days. Cells were then collected and fixed in 1% PFA + 1× protease inhibitor cocktail (PIC) for 10 min followed by quenching for 10 min with 0.125 M glycine. Cells were washed and sonicated to 100–500 bp fragments. Chromatin complexes were incubated with antibodies (Supplementary Table 1 ) overnight at 4 °C. Antibodies/chromatin complexes were captured on magnetic Protein A Dynabeads (Invitrogen) for 4 h followed by washing and elution. Chromatin complexes were then reverse cross-linked for 12–16 h at 65 °C. Chromatin was cleaned using the Qiagen PCR purification kit. 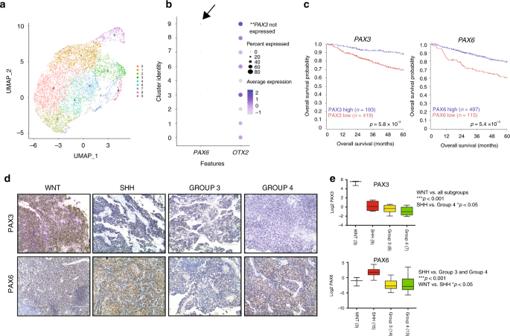Fig. 2: PAX3 and PAX6 protein levels are lower in Group 3 MB, and lower expression of both genes is associated with reduced survival in patients. aNine transcriptionally distinct cell populations from two Group 3 MB patient samples as previously defined11. Of note, clusters 5, 10, and 11 were classified as non-tumor clusters and removed for downstream analysis.bDot plot demonstrating the frequency and average expression ofPAX6(left) andOTX2(right) within nine transcriptionally distinct cell populations fromN= 2 Group 3 MB patient samples. Arrow denotes minimal expression ofPAX6in cluster 9.PAX3was not detected in this dataset.cLow expression of bothPAX3andPAX6is associated with significantly reduced overall patient survival inN= 612 MB patient samples.p-Values were determined using the log-rank method.dRepresentative images of PAX3 and PAX6 staining in FFPE sections from all four MB subgroups. Scale = 200 μm.eProteomic analysis (Boston cohort) demonstrates low expression of PAX3 (N= 27 patient samples) and PAX6 (N= 45 patient samples) in Group 3 MB. For PAX3: WNT vs all other subgroups, ***p< 0.001, SHH vs Group 4: *p< 0.05, all other pairs NS. For PAX6: WNT vs SHH, *p< 0.05, SHH vs Group 3 and Group 4 ***p< 0.001, all other pairs NS. Significance was determined by one-way ANOVA. For ChIP-qPCR, chromatin was amplified with appropriate primers (Supplementary Table 2 ), and fold enrichment of protein binding was calculated and graphed with Prism 8.0. ChIP-sequencing reads were trimmed using Trimmomatic 0.36 [52] . The resulting trimmed sequences were mapped to GRCh38 using bowtie2 2.3.3.1 [53] . Histone differential peak analysis was performed using diffReps [54] . G-test comparisons were performed in “block” mode for H3K27me3 and in “peak” mode for H3K4me3, utilizing the OTX2 high and low input samples treatment group backgrounds. Enriched regions were associated with Ensembl GRCh38 annotations downloaded using BioMart [55] . Based on this integrated data, genes containing diffReps identified H3K4me3 differentially enriched regions in the −5 kb to +2 kb regions around the TSS and H3K27me3-enriched regions over the gene body were generated, and the gene list submitted to Ingenuity Pathway Analysis ( https://www.qiagenbioinformatics.com/products/ingenuity-pathway-analysis ) to determine enriched pathways and Gene Ontology terms. In addition, OTX2 motifs were identified in OTX2 peaks [25] using the following motif patterns (TCTAATCCC, TAATCC, TAAGCC, TAATCT, TAACCC) available as a part of the publication UCSC track hub ( http://dropbox.ogic.ca/trackhubs/ogilvie/hub.txt ). For patient histone ChIP-sequencing data [22] , the GEO series GSE92585 provided wiggle files of mean read depth over 25 bp windows across the genome. The original GEO wiggle files were mapped to GRCh37; we performed a liftover to GRCh38 and normalized the resulting wiggle files to reads per million. Plots were scaled on the y -axis based on the maximum normalized H3k4me3 and H3k27me3 values, respectively, for OTX2 , PAX3 , and PAX6 . Co-immunoprecipitation Group 3 MB cells were grown in stem cell conditions for 3 days and dissociated into a single-cell suspension. Cells were immediately lysed with IP lysis buffer (25 mM Tris pH7.4, 150 mM NaCl, 1% Triton X-100, 5 mM EDTA) plus 1× PIC. Samples were precleared for 2 h with rotation at 4 °C. Immunoprecipitation was carried out overnight with 2 μg of IgG or OTX2 antibody. Magnetic beads were blocked with 1% BSA solution for 1 h, washed and then added to the antibody/protein complexes for 3 h with rotation at 4 °C. Beads were then washed 5X with IP lysis buffer. Complexes were eluted from the beads by boiling for 5 min in 1× SDS sample buffer. Protein–protein interaction was then determined by immunoblotting as described below. siRNA silencing OTX2 expression was silenced in Group 3 cells using Silencer Select siRNAs 9931 and 9931 (Life Technologies) at 30 nM concentrations. Scramble non-silencing siRNA was utilized as a negative control. OTX2 knockdown was validated by western blot. Patient transcriptome and proteomic analysis PAX3 and PAX6 expression was analyzed in 763 subtyped primary MB samples previously profiled on the Affymetrix Gene 1.1ST arrays [5] and normalized using the RMA method. Primary samples were subtyped by similarity network fusion (GSE85217). For analyses, ANOVA in the R statistical environment (v3.4.2) was used to evaluate differences across subgroups and subtypes. Survival was measured from initial diagnosis to death or last follow-up and estimated using parameters described in both the Cavalli et al. and Cho et al. datasets [5] , [56] . p < 0.01 were significant. The Cavalli et al. 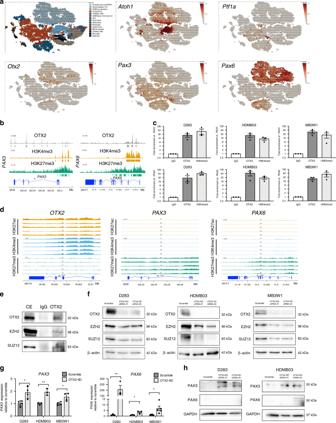Fig. 3: OTX2 directly regulates the expression ofPAX3andPAX6in Group 3 MB. aScatterhex plots showing expression of select genes obtained fromhttps://cellseek.stjude.org/cerebellum/. The gene expression of a hexgrid is summarized as the mean expression of all component cells and compared with predicted cell type mapped onto the scatterhex grid (upper left).bOTX2 enrichment is observed at regulatory elements onPAX3andPAX6, overlapping with H3K4me3 and H3K27me3 bivalency marks.cOTX2 binding toPAX3andPAX6was validated in D283, HDMB03, and MB3W1 Group 3 MB tumorspheres by ChIP-qPCR. Data are presented as mean values ± SEM.N= 3 biological replicates for each cell line. H3K4me3 ChIP-qPCR was used as a positive control.dEnrichment of H3K4me3, H3K27ac, and H3K27me3 at regulatory elements ofOTX2,PAX3, andPAX6, respectively, in five Group 3 MB patient samples as originally defined by Boulay et al.eCo-immunoprecipitation experiments showing protein–protein interaction between OTX2 and EZH2/SUZ12 in HDMB03 tumorspheres. CE cellular extracts.fEZH2 and SUZ12 levels are reduced following OTX2 silencing in D283, HDMB03, and MB3W1 tumorspheres. β-actin serves as the loading control.gPAX3(left) andPAX6(right) expression are significantly increased in Group 3 MB tumorspheres following OTX2 silencing for 72 h. Data are presented as mean values ± SEM and plotted as fold expression relative to scramble control.N= 3 biological replicates (PAX3expresion in HDMB03,PAX6expression in D283, HDMB03);N= 4 biological replicates (PAX3expression in D283, MB3W1); orN= 5 biological replicates (PAX6expression in MB3W1). Significance was determined using an unpaired two-tailedt-test for each pair. ForPAX3: D283p= 0.015; HDMB03p= 0.005; MB3W1p= 0.016. ForPAX6: D283p= 0.005; HDMB03p= 0.041; MB3W1p= 0.023.hPAX3, but not PAX6 levels are increased following OTX2 silencing in D283 and HDMB03 tumorspheres. GAPDH serves as the loading control. dataset [5] was also subjected to pathway enrichment analyses. Group 3β and 3γ MB samples were tested for differentially expressed genes against the rest of the subgroups using edgeR [57] . Rank for each gene was constructed using the log-fold change multiplied by log of p -values of the gene as obtained through edgeR analysis. Further, the ranked list was subjected to preranked GSEA analysis [58] . A q -value of 0.25 was considered significant for the pathways and network was constructed using Enrichmentmap app [59] in Cytoscape v3.7.2 [60] . Protein levels of OTX2, PAX3, and PAX6 were assessed using available proteomics data from human MBs [37] , [61] . PAX3 protein levels were only detected in the Tenley et al. dataset; therefore, this dataset was used for subsequent analysis. Box plots were generated using the GraphPad Prism software and one-way ANOVA was performed using the Partek® Genomics Suite® software. Analysis of single-cell cerebellar murine transcript data Scatterhex plots showing expression of select genes were obtained from https://cellseek.stjude.org/cerebellum/ . This website enables interactive exploration of recently published single-cell transcription profiles generated throughout murine cerebellar development [38] . The gene expression of a hexgrid is summarized as the mean expression of all component cells and this is compared with predicted cell type mapped onto the scatterhex grid. Quantitative real-time PCR Whole RNA was extracted from Group 3 MB cells using a Norgen-all-in-one kit (Norgen Biotek, Thorold, ON, Canada). The Superscript III First Strand Synthesis kit (Life Technologies) was used for first-strand cDNA synthesis. qPCR was performed using the GoTaq qPCR Master Mix (Fisher Scientific, Ottawa, ON, Canada) and data were analyzed on a Mx3000 P Stratagene qPCR system, using the following parameters: 50 °C for 2 min, 95 °C for 2 min, and 40 cycles of 95 °C for 15 s and 60 °C for 30 s. Primer sequences for each specific gene evaluated are listed in Supplementary Table 2 and values were normalized to GAPDH . PAX GOF lentiviral transduction HDMB03 cells were plated at 4 × 10 5 cells/well in tumorsphere forming conditions as described above. Dharmacon (Chicago, IL, USA) Precision LentiORF PAX3 (OHS5836-EG5077), PAX6 (OHS5899-202618462), or RFP control lentiviral particles were added to the cells 24 h following seeding at MOI = 0.3. The following day, lentiviral particles were removed and fresh tumorsphere media was added. Selection of positively transduced cells was carried out 72 h after infection with 25 μg/mL blasticidin. RNA sequencing and analyses Whole RNA was extracted from PAX GOF tumorspheres using the Norgen RNA extraction kit (Norgen Biotek). Library preparation and RNA sequencing (RNA-seq) were performed by StemCore laboratories at the Ottawa Hospital Research Institute (Ottawa, ON, Canada). RNA-seq reads were mapped to transcripts from GENCODE release 27 using salmon v0.9.1 [62] between 83 and 89% of reads in each sample were assigned to transcripts from the GENCODE v.27 assembly. Data were loaded into R using the tximport library, and the gene/count matrix was filtered to retain only genes with five or more mapped reads in two or more samples. Differential expression was assessed using DESeq2 (v1.20.0) [63] comparing three conditions (control, PAX3 GOF, and PAX6 GOF). Principal component analysis (PCA) was performed using the DESeq2 plotPCA function, and hierarchical clustering was run using Euclidian distance; both using rlog- transformed count data. Expression differences between control and PAX3 GOF or PAX6 GOF were calculated using the lfcShrink function, applying the apeglm method (v 1.2.1) [64] . Lists of significantly changed genes were identified using a q -value (Benjamini–Hochberg corrected p -value) cutoff of 0.05. Lists of genes with significant positive and negative fold changes for PAX3 GOF and PAX6 GOF were subjected to functional enrichment analysis, using the clusterProfiler (v3.8.1) package [65] in R. Over-enrichment was calculated for GO Biological Process and Molecular Functional annotations in lists of genes (a) significantly higher in PAX3 GOF than in control (b) significantly lower in PAX3 GOF than in control (c) significantly higher in PAX6 GOF than in control (d) significantly lower in PAX6 GOF than in control. GSEA [58] was run using preranked gene lists (the GSEA preranked method) to explore enrichment of pathways and functional classes in the genes, with the most significantly changed expression in PAX3 and PAX6 GOF samples. The gene lists for PAX3 and PAX6 GOF were filtered to retain protein-coding genes, and ranked by fold change confidence using the function “ -log10(p-value)*sign(log2FoldChange) ”. GSEA was run using the MSigDb (v6.1) [66] collections H (hallmark gene sets), C2:CP (canonical pathways), and C6 (oncogenic signatures). Single-cell cDNA library generation and RNA sequencing Single-cell cDNA libraries were generated using the 10× Genomics Single Cell 3′ Reagents Kits v3 and Chromium controller. HDMB03, D283, and MB3W1 tumorspheres were dissociated into single-cell suspensions and assessed for cell viability. HDMB03, D283, and MB3W1 single-cell suspensions were then resuspended in 0.04% BSA in 1× PBS at a cell concentration of 1200 live cells per µl to achieve a targeted cell recovery of 6000 cells per sample. Quality control of the 10× Genomics-indexed cDNA libraries were performed on the 2100 Bioanalyzer (Agilent Technologies) and Qubit 4 Fluorometer (Thermo Fisher Scientific). Then, 4 nM each of the HDMB03, D283, and MB3W1 cDNA libraries were pooled together, and sequenced on a NextSeq 500 at StemCore laboratories (Ottawa, ON, Canada) to generate the recommended UMI and transcript reads (28 bp and 55 bp, respectively). Single-cell RNA-seq analysis 10× Genomics libraries generated from HDMB03, D283, and MB3W1 tumorspheres were processed with 10× Cellranger software to generate count matrices, using the standard 10× GRCh38 reference (v3.0.0). Matrices were loaded into the R package Seurat (v3.0.0) for analysis and filtered to remove cells with high mitochondrial content (9% mitochondrial UMIs for D283, 32% for HDMB03, and 11% for MB3W1) and low RNA counts (<200 features). Data were normalized and variable features identified, followed by data scaling and dimensionality reduction by PCA using the identified variable genes. Differences between the G2M and S phase scores were regressed out to maintain signals separating non-cycling and cycling cells, using Seurat CellCycleScoring and ScaleData functions. 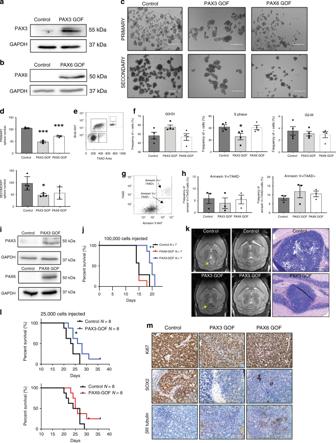Fig. 4: Increased PAX3 and PAX6 expression reduces tumorigenic properties of Group 3 MB cells. a,bPAX3 (a) and PAX6 (b) overexpression in HDMB03 Group 3 MB tumorspheres. GAPDH serves as the loading control.c,dRepresentative images (c) and quantification (d) of primary and secondary tumorspheres, with increased expression of PAX3 and PAX6. Error bars: SEM. Scale = 200 μm.N= 3 biological replicates for primary tumorspheres andN= 4 biological replicates for secondary tumorspheres. Significance was determined by ANOVA and a Tukey’s test for multiple comparisons. For primary tumorspheres: PAX3 GOF,p< 0.0001; PAX6 GOF,p= 0.0004. For secondary tumorspheres: PAX3 GOF,p= 0.023.e,fBrdU incorporation analysis in PAX3 and PAX6 GOF cells. Representative dot plot of gating strategy for BrdU analyses with 7AAD only control (inset) (e) and quantification of cell cycle phases in control, PAX3 GOF, and PAX6 GOF tumorspheres (f). Data are presented as mean values ± SEM. For PAX3 GOF “S” phase,p= 0.043.N= 4 biological replicates.g,hAnnexin V/7AAD analyses of cell viability in PAX3 and PAX6 GOF cells. Representative dot plot of gating strategy for Annexin V/7AAD analyses (g) and quantification of live/dead cells in control, PAX3, and PAX6 GOF tumorspheres (h). Data are presented as mean values ± SEM.N= 3 biological replicates. For all flow cytometry data, signficance was determined by ANOVA followed by a Dunnett for multiple comparisons.iIncreased PAX3 (upper) and PAX6 (lower) expression in HDMB03 cells utilized for intracerebellar transplants. GAPDH serves as the loading control.jKaplan–Meier curves depicting overall survival in animals transplanted with 1 × 105control, PAX3, or PAX6 GOF cells.p-Values determined using the log-rank method andp= 0.0014.kMRIs from two independent control and PAX3 GOF tumors (left) and H&E staining (right) from control and PAX3 GOF xenografts. Arrows denote tumors in the cerebellum. Scale = 400 μm.lSurvival in xenografts transplanted with 2.5 × 104control, PAX3, or PAX6 GOF cells.p-Values determined using the log-rank method andp= 0.040.mRepresentative images of Ki67, SOX2, and βIII tubulin levels in control, PAX3, and PAX6 GOF HDMB03 MB tumor-bearing mice. Scale bar: 100 μm. Cells were clustered using an SNN modularity optimization method on the first 15 principal components (Seurat FindNeighbors and FindClusters functions), and data visualized using a Uniform Manifold Approximation and Projection (UMAP) projection. Cluster markers were identified using Seurat’s FindAllMarkers function. Integration was performed using harmony package [67] with default parameters, and using sample ID as a variable to regress out. We then clustered cells using an SNN modularity optimization method on the harmony embeddings with standard deviation >3.5 (elbow). Data were visualized using a UMAP projection. For analyses of patient samples, filtered gene matrices from two Group 3 MB tumors were downloaded from the European Genome-phenome Archive (EGA portal: EGAS00001003170 ) [11] . Cells with at least 1000 genes expressed and a mitochondrial content below the 75th percentile + 3 × IQR were loaded into R package Seurat (version 3.0.0) for clustering analysis. Signal from cell cycle genes has been regressed out using CellCycleScoring function from Seurat. Data were normalized according to SCTransform function. Data integration were performed using RunHarmony implemented in Seurat to perform batch correction and meta-analysis. Linear dimensionality reduction was performed using PCA [11] , and the top ten principal components were selected according to the elbow plot [11] . A Shared Nearest Neighbor (SNN) modularity optimization-based clustering algorithm was used to perform cell clustering and visualization was performed using UMAP. Based on their most differentially expressed genes [11] clusters 5, 10 and 11 were classified as non-tumor clusters and removed for downstream analysis. Immunohistochemistry FFPE tissue from surgically resected MB patient samples was obtained with informed consent and following the ethical regulations at the University of Manitoba, the Hospital for Sick Children and the University of Calgary’s Clark Smith Brain Tumour Bank. MB subgroup classification was previously determined by NanoString profiling analyses [68] . Following deparaffinization of FFPE patient or xenograft samples, antigen retrieval was performed in citrate buffer at 95–100 °C for 20 min. Slides were washed and treated for 10 min for endogenous peroxidase, and again washed in 1× PBS. The samples were blocked with 3% lamb serum, then incubated with primary antibodies (Supplementary Table 1 ) overnight at 4 °C. Slides were treated with secondary antibody (Supplementary Table 1 ) for 2 h at room temperature. Streptavidin/HRP (Jackson ImmunoResearch, West Grove, PA, USA) in 1× PBS was then added for 30 min followed by development with DAB and counterstaining with hematoxylin. Finally, coverslips were mounted with Permount (Fisher Scientific). BrdU and Annexin V analysis BrdU incorporation and cell cycle analyses were performed with a BD Pharmingen BrdU Flow Kit (BD Biosciences), following manufacturer’s guidelines in PAX GOF tumorspheres grown for 72 h in stem cell conditions. The Annexin V Apoptosis Detection Kit (BD Biosciences) was used to evaluate cell death following manufacturer’s guidelines. Dissociated PAX GOF tumorspheres were stained with Annexin V, followed by 7AAD. 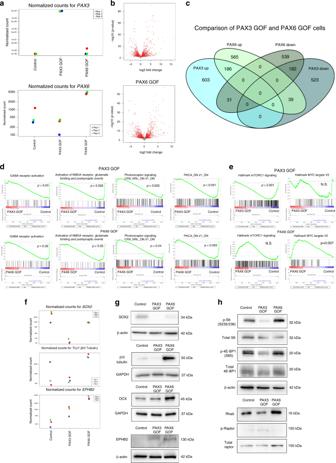Fig. 5: PAX3 and PAX6 expression perturb Group 3 transcriptional signatures. aIncreased expression ofPAX3andPAX6in Group 3 HDMB03 PAX3 and PAX6 GOF tumorspheres validated at the transcript level by RNA sequencing.bVolcano plots depicting fold changes of differentially expressed genes identified in PAX3 (1564) and PAX6 (1542) GOF tumorspheres. *p< 0.05 for all genes.cVenn diagram comparing unique and shared upregulated or downregulated genes identified to be differentially expressed in PAX3 and PAX6 GOF HDMB03 tumorspheres. *p< 0.05 for all genes.dGSEA demonstrating that GABA receptor activation, as well as glutamate and PKCA signaling are enriched in gene sets that are downregulated in PAX3 and PAX6 GOF tumorspheres. Genes associated with photoreceptor signaling are enriched in gene sets that are commonly upregulated in PAX3 and PAX6 GOF tumorspheres.emTORC1 signaling is enriched in gene sets that are downregulated in PAX3 GOF tumorspheres. Genes associated with MYC targets are enriched in PAX6 GOF tumorspheres.fNormalized cell counts from RNA sequencing data showing decreasedSOX2, and increasedTUJ1(βIII tubulin) orEPHB2in PAX3 and/or PAX6 GOF tumorspheres.gValidation of changes in SOX2, βIII tubulin, EPHB2, and DCX levels in PAX GOF tumorspheres. β-actin and GAPDH serve as loading controls.hReduction in overall mTORC1 activity output observed specifically in PAX3 GOF tumorspheres. Total S6, total 4E-BP1, total Raptor, and β-actin serve loading controls. Note that for all RNA sequencing data, significantly different genes were identified using aq-value (Benjamini–Hochberg correctedp-value) cutoff of 0.05. Samples were run on a MoFlo XDP cell sorter (Beckman Coulter, Mississauga, ON, Canada) and analysis was performed using Kaluza software (Beckman Coulter). Immunoblotting Protein quantities ranging from 10–25 μg were loaded onto 10–12% Tris-glycine gels and resolved by SDS–PAGE. Protein was transferred to nitrocellulose membranes and blocked with 5% milk. Membranes were incubated overnight at dilutions outlined in Supplementary Table 1 . Secondary antibodies conjugated to horseradish peroxidase were added the following day for 1 h at room temperature, and then detected using SuperSignal West Pico. Images were captured on a Fusion FX Vilber Lourmat chemiluminescent imaging system (Marne-la-Vallee cedex 3, France). Intracerebellar transplantation and drug treatment The University of Manitoba’s Animal Care Committee approved all procedures. Group 3 MB tumorspheres were dissociated and 1 × 10 5 or 2.5 × 10 4 cells were injected into the cerebellums of 7–9-week-old NOD-SCID mice. NOD-SCID mice were housed in IVC caging (Tecniplast) and held according to the Guidelines of the Canadian Council on Animal Care and the Animal Care and Use Policy of the University of Manitoba. Irradiated feed was used and caging and bedding were sterilized by steam autoclave. Room ambient temperature was 21–23°C with a relative humidity target of 50%, but within a range of 30–60%. Light cycle was 12 h on/12 h off beginning with lights on at 6:00 a.m. Animals were perfused with formalin after a reduction of 20% of peak body weight was observed or after 12–14 days to assess growth differences. MRI of PAX3 GOF tumors was performed using a MR Solutions cryogen free FlexiScan 7 T system (MR Solutions, Guildford, Surrey, UK). Brains were extracted and placed in formalin for 5–7 days prior to processing for histopathology. For PQR620 drug treatments, all mice were injected with 1 × 10 5 (HDMB03) cells. At day 5, animals were randomly separated and received either PQR620 at 50 or 100 mg/kg or 0.5% hydroxypropyl methyl cellulose, 0.1% polysorbate 80 + 2% HCl as the vehicle control. PQR620 was administered twice daily, 5 days a week, via oral gavage until endpoint was reached as described above. Statistical analysis Prism 8.0 software (GraphPad Software) was used to analyze all data. Tumor survival was evaluated using the log-rank (Mantel–Cox) method. All in vitro data were assessed by one-way ANOVA followed by a Dunnett test or Tukey’s test for multiple comparisons as appropriate. Homogeneity of variances was assessed using a Brown–Forsythe test. p ≤ 0.05 were considered significant. 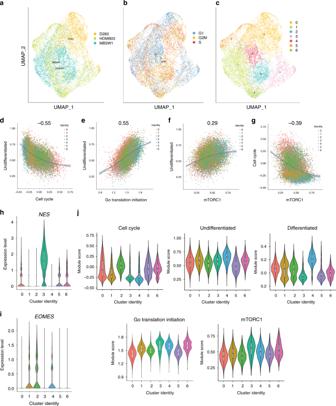Fig. 6: Integrated scRNA-seq analyses of Group 3 tumorspheres reveals relationships between the undifferentiated stem/progenitor cell state and an mTORC1 gene expression signature. a–cUMAP representations of integrated tumorsphere data from D283, HDMB03, and MB3W1 (a), cell cycle phases from integrated data (b), and transcriptionally distinct cell populations from integrated data (c).d–gCorrelation plots displaying the relationship between the undifferentiated program and cell cycle (d), as well as the undifferentiated program and translation initiation (e), the undifferentiated program and our mTORC1 gene signature (f), and cell cycle and our mTORC1 gene signature (g) from integrated tumorsphere data. The mTORC1 gene signature overlaps with the broad translation initiation program, but is based on the curated list of genes provided in Supplementary Data8, the majority of which  are associated with the 4E-BP1 and S6 ribosomal protein arms of mTORC1 signaling, and are also direct OTX2 targets.h,iExpression of the neural stem cell marker Nestin (NES) and the differentiated unipolar brush cell marker Eomesodermin (EOMES) in clusters of the integrated tumorsphere data.jExpression of the cell cycle, undifferentiated, differentiated, and translation initiation programs, as well our mTORC1 gene expression signature across clusters in the integrated tumorsphere data. For the three biologically independent cell lines,n= 6307 cells (HDMB03),n= 5297 cells (D283), andn= 5099 cells (MB3W1). For all violin plots, the center line is the median, the 25th and 75th percentiles are depicted by the bottom and top of the box, respectively, and the whiskers extend to the minima and maxima. 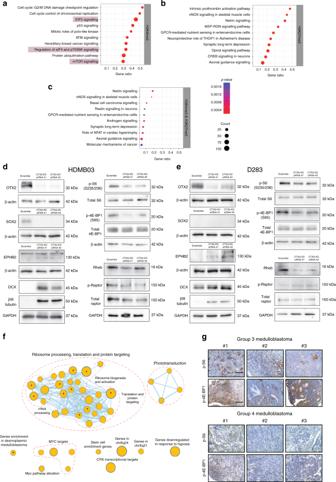Fig. 7: Loss of OTX2 phenocopies PAX3 and PAX6 GOF in Group 3 MB cells. a–cEIF2 and mTORC1 signaling (highlighted) associated with genes that have significant changes in the H3K4me3 modification, following OTX2 silencing in Group 3 MB tumorspheres. Significance was calculated using a right-tailed Fisher’s exact test.d,eOTX2 silencing in HDMB03 (d) and D283 (e) tumorspheres with two independent siRNAs reduces SOX2, p-S6, p-4E-BP1, and Rheb levels. The neuronal differentiation markers DCX, βIII tubulin, and EPHB2 are increased along with small increases in pRaptor in D283 tumorspheres only. Total S6, total 4E-BP1, total Raptor, GAPDH, and β-actin serve as loading controls.fEnriched biological processes and pathways determined using GSEA (Terms with FDR correctedq-value < 0.25) and visualized in Cytoscape v3.7.2 using Enrichmentmap. Each node in the map denotes a pathway, process or a transcription factor enrichment. The size of the nodes is proportional to the number of genes in the process. The nodes are connected when they share enriched genes. Nodes with asterisk denote the processes enriched withq< 0.05.gRepresentative images of p-S6 and p-4E-BP1 immunohistochemical staining in three independent FFPE Group 3 (upper) and Group 4 (lower) MB patient samples. Scale = 200 μm. 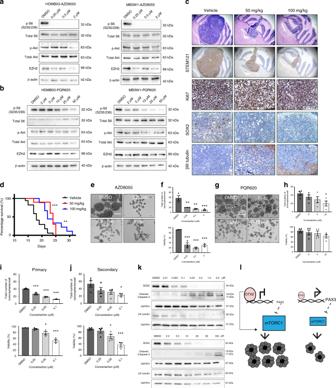Fig. 8: mTORC1 signaling regulates tumorsphere formation and self-renewal in Group 3 MB. a,bmTOR signaling and EZH2 levels following 3 h AZD8055 (a) or 24 h PQR620 (b) treatment in Group 3 MB tumorspheres. Total S6, total AKT, and β-actin serve loading controls.cRepresentative H&E as well as immunohistochemical images of STEM121, Ki67, SOX2, and βIII tubulin levels in control and PQR620-treated HDMB03 tumor-bearing NOD-SCID mice 14 days postinjection. Scale bars: 1000 μm (H&E and STEM121) or 100 μm (Ki67, SOX2, βIII tubulin).dSurvival in animals transplanted with 1 × 105cells from HDMB03 tumorspheres and treated with vehicle (N= 17) or PQR620 (N= 10 50 mg/kg, andN= 9 100 mg/kg).p-Value determined using the log-rank method.p= 0.0001 for 50 mg/kg andp= 0.002 for 100 mg/kg.eRepresentative images of tumorspheres following AZD8055 treatment of HDMB03 Group 3 MB cells. Scale = 200 μm.fQuantification of total sphere number (upper) and viability (lower) following HDMB03 Group 3 tumorsphere treatment with AZD8055. Error bars: SEM.N= 3 biological replicates. For total sphere number:p= 0.0035 (0.25 μM);p= 0.0014 (0.5 μM);p= 0.0007 (2.0 μM). For viability:p< 0.0001 for all concentrations.gRepresentative images of tumorsphere number following HDMB03 PQR620 treatment. Scale = 200 μm.hQuantification of total sphere number (upper) and viability (lower) following HDMB03 treatment with PQR620.N= 4 biological replicates. For total sphere number:p= 0.038 (10 μM).i,jQuantification of primary (i) and secondary (j) HDMB03 tumorsphere number, and viability following AZD8055 treatment (25–100 nM). For primary sphere number:p= 0.002 (0.025 μM);p< 0.0001 for remaining concentrations. For viability:p= 0.0362 (0.05 μM);p= 0.0002 (0.1 μM). For secondary sphere number:p= 0.043 (0.1 μM). For viability:p= 0.035 (0.05 μM);p= 0.0004 (0.1 μM).kWestern blots depicting SOX2, βIII tubulin, and cleaved caspase 3 levels, following AZD8055 (upper) or PQR620 (lower) treatment of HDMB03 tumorspheres at 24–72 h. GAPDH serves as the loading control. For all tumorsphere studies, data are presented as mean values ± SEM, and significance was determined by one-way ANOVA and a Dunnett test for multiple comparisons.lModel demonstrating an OTX2-PAX3 circuitry regulates cell fate decisions through control of mTORC1 signaling. All data reported as ±SEM. Reporting summary Further information on research design is available in the Nature Research Life Sciences Reporting Summary linked to this article.